Insertion sequence-excision enhancer removes transposable elements from bacterial genomes and induces various genomic deletions Insertion sequences (ISs) are the simplest transposable elements and are widely distributed in bacteria. It has long been thought that IS excision rarely occurs in bacterial cells because most bacteria exhibit no end-joining activity to regenerate donor DNA after IS excision. Recently, however, we found that excision of IS 629 , an IS 3 family member, occurs frequently in Escherichia coli O157. In this paper, we describe a protein IS-excision enhancer (IEE) that promotes IS 629 excision from the O157 genome in an IS transposase-dependent manner. Various types of genomic deletions are also generated on IEE-mediated IS excision, and IEE promotes the excision of other IS 3 family members and ISs from several other IS families. These data and the phylogeny of IEE homologues found in a broad range of bacteria suggest that IEE proteins have coevolved with IS elements and have pivotal roles in bacterial genome evolution by inducing IS removal and genomic deletion. Transposable elements (TEs), or transposons (Tns), are widely distributed in eukaryotic and prokaryotic genomes. They are considered selfish (or parasitic) genetic elements, but they also have important roles in genome evolution [1] . Insertion sequence (IS) elements, which are the simplest TEs, are 700–2,500 bp in size and encode only the transposase (TPase) catalysing their own transposition [2] . The transposition and proliferation of IS elements induce not only insertional gene inactivation and modification of gene expression [1] but also a variety of genomic rearrangements, such as deletions, inversions and duplications [3] , [4] . In bacteria, several thousand types of IS elements have thus far been identified from various species and strains [5] . These elements are classified into ∼ 20 families on the basis of the sequences of their TPases and terminal inverted repeats (TIRs), in addition to several other features [2] . The mechanism of transposition differs between IS families, but IS elements transpose and either leave the original copy in the donor DNA (termed copy-and-paste, or replicative, transposition) or eradicate it from the donor DNA (cut-and-paste, or non-replicative, transposition) [6] . The mechanisms of transposition have been intensively studied for representative IS elements of several families, and one of the best studied is the IS 3 family. The process of transposition in this large IS family is initiated by the formation of a 'figure-eight intermediate,' which is followed by the generation of an excised circular DNA molecule that is randomly inserted into the target DNA [2] . Although the entire process is not yet fully understood at the molecular level, it has been demonstrated for IS 911 , a representative family member, that a replicative pathway is used to generate a circular DNA molecule from the figure-eight intermediate. Thus, IS 911 transposes by the copy-and-paste mechanism [7] . If the copy-and-paste mechanism is the major pathway for the transposition of the IS 3 family, the excision of IS 3 family members occurs very rarely in the normal transposition process. In general, researchers believe that the excision of IS elements is a rare genetic event in bacteria [8] , because end-joining systems, which are required to reseal the donor DNA for its survival after IS excision, have been identified in relatively few bacterial species [9] . Thus, very little attention has been paid to the genetic events that occur to donor DNA on IS excision. Tn excision in bacteria has been described in several reports, but such excision was observed to be independent of TPase activity. Instead, it is dependent on host factors required for replication slippage and repair functions [10] , [11] . In practise, these excision events have been observed at a low frequency. However, we recently obtained several lines of evidence to show that excision of IS 629 , a member of the IS 3 family, occurs frequently in the enterohaemorrhagic Escherichia coli (EHEC) strain O157. EHEC O157 produces highly potent cytotoxins (Shiga toxins Stx1 and/or Stx2) and causes diarrhoea, haemorrhagic colitis and haemolytic uremic syndrome, thus being regarded as one of the most serious worldwide food-borne infections [12] . The O157 strain that has been sequenced (RIMD0509952, referred to as O157 Sakai) contains 25 types of IS elements (116 copies in total) [13] . Among these elements, the most abundant is IS 629 (also called IS 1203 v): 23 copies are present on the bacterial chromosome and on the pO157 virulence plasmid. Of these copies, 17 (74%) are apparently intact, whereas only 22 copies (24%) are intact among other types of IS elements, suggesting that active copies of IS 629 are selectively maintained in EHEC O157. In fact, our comparative genomic analysis of EHEC O157 clinical isolates revealed that many small-sized structural polymorphisms associated with gene inactivation and/or deletion have been generated by IS 629 in EHEC O157 strains [14] . Several genomic loci in which IS 629 has been deleted by simple excision were also identified. In another series of studies, we observed that an stx2 gene that was inactivated by IS 629 insertion, which was found in some O157 clinical isolates [15] , [16] , was reactivated by precise IS 629 excision in the E. coli laboratory strain K-12 (but at a very low frequency) [17] . However, using a reporter plasmid-based assay, we found that precise IS 629 excision occurs much more frequently in O157 Sakai than in K-12, and several other EHEC strains also exhibit a high frequency of IS 629 excision [18] . These results suggest that some E. coli strains, including O157, may contain a previously unknown system to promote IS excision by regenerating the donor DNA lacking the IS copy. The clear difference between O157 Sakai and K-12 in excision frequency further suggests that this system may be encoded by one or more of the ∼ 1,600 O157 Sakai genes that are not present in K-12 (ref. 19 ). Here, we describe an O157 Sakai gene that promotes the excision of IS 629 and of several other ISs in a TPase-dependent manner and generates various types of genomic deletions on IS excision, thus having a pivotal role in bacterial genome evolution. We further identify many homologues of this gene, which appear to have been spread by horizontal gene transfer and to have been coevolved with IS elements, in a wide range of bacteria. Identification of a protein that enhances IS 629 excision To identify a genetic determinant(s) that is responsible for a high frequency of IS 629 excision in O157 and other EHEC strains, we first analysed, using a reporter plasmid ( Fig. 1a ), the frequencies of precise IS 629 excision in K-12, O157 Sakai and 13 other EHEC strains of the O157, O26, O111 or O103 serotype, the whole gene repertoires of which were previously analysed by comparative genomic hybridization using an O157 oligo DNA microarray [20] . Among the 15 strains tested, 11 EHEC strains (including O157 Sakai) exhibited a high excision frequency, whereas 4 strains (O157 #3, O26 #1, O103 #6 and K-12) showed no or an extremely low excision frequency ( Fig. 1b ). By reinspecting the comparative genomic hybridization data for these 15 strains, we found that ECs1305, which encodes a hypothetical protein, was the only gene that was present in the high frequency group but not in the low frequency group. 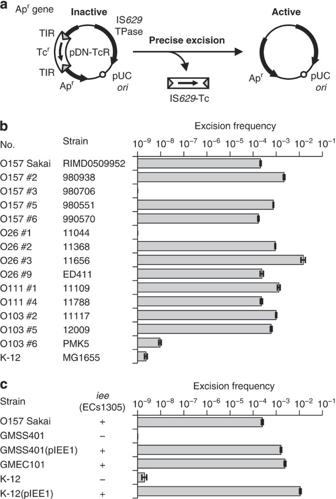Figure 1: IS629excision frequencies in variousE. colistrains. (a) Schematic representation of the reporter plasmid assay for analysing the frequency of the precise excision of IS629. (b) Frequencies of precise IS629excision in K-12, O157 Sakai and another 13 EHEC strains of O157, O26, O111 and O103 serotypes. The excision frequency was determined using the reporter plasmid assay shown in panel (a) and calculated by dividing the number of ampicillin-resistant (Apr) colonies by that of tetracycline-resistant (Tcr) colonies (mean±s.d.,n=3). Four strains (O157 #3, O26 #1, O103 #6 and K-12) exhibited radically lower excision frequencies (<10−7) compared with the other 11 strains (>10−4), which included O157 Sakai. No Aprcolonies were obtained for O157 #3 or O26 #1. (c) The effects of ECs1305 (theieegene) on IS629excision frequency in O157 Sakai, K-12 and their derivatives. ECs1305 is encoded by a large integrative element called SpLE1 in the genome of O157 Sakai. GMSS401 is aniee-deletion mutant of O157 Sakai. GMEC101 is a K-12 derivative in which theieegene was inserted into an IS3copy on the chromosome. GMSS401(pIEE1) and K-12(pIEE1) contain a plasmid carrying theieegene. The excision frequency was determined as in panel (b). Plus and minus symbols indicate the presence and absence of theieegene in each strain, respectively. No Aprcolonies were obtained for GMSS401. Figure 1: IS 629 excision frequencies in various E. coli strains. ( a ) Schematic representation of the reporter plasmid assay for analysing the frequency of the precise excision of IS 629 . ( b ) Frequencies of precise IS 629 excision in K-12, O157 Sakai and another 13 EHEC strains of O157, O26, O111 and O103 serotypes. The excision frequency was determined using the reporter plasmid assay shown in panel ( a ) and calculated by dividing the number of ampicillin-resistant (Ap r ) colonies by that of tetracycline-resistant (Tc r ) colonies (mean±s.d., n =3). Four strains (O157 #3, O26 #1, O103 #6 and K-12) exhibited radically lower excision frequencies (<10 −7 ) compared with the other 11 strains (>10 −4 ), which included O157 Sakai. No Ap r colonies were obtained for O157 #3 or O26 #1. ( c ) The effects of ECs1305 (the iee gene) on IS 629 excision frequency in O157 Sakai, K-12 and their derivatives. ECs1305 is encoded by a large integrative element called SpLE1 in the genome of O157 Sakai. GMSS401 is an iee -deletion mutant of O157 Sakai. GMEC101 is a K-12 derivative in which the iee gene was inserted into an IS 3 copy on the chromosome. GMSS401(pIEE1) and K-12(pIEE1) contain a plasmid carrying the iee gene. The excision frequency was determined as in panel ( b ). Plus and minus symbols indicate the presence and absence of the iee gene in each strain, respectively. No Ap r colonies were obtained for GMSS401. Full size image We detected no precise IS 629 excision in an ECs1305-deletion mutant of O157 Sakai (strain GMSS401 in Fig. 1c ), and the excision frequency of the mutant returned to the parental level by reintroducing ECs1305 (GMSS401(pIEE1)). Furthermore, K-12 derivatives containing ECs1305 (chromosomally inserted or plasmid encoded) showed a high IS 629 excision rate comparable to or higher than that in O157 Sakai (GMEC101 and K-12(pIEE1) in Fig. 1c ). These results indicate that ECs1305 enhances precise IS 629 excision in the genetic backgrounds of O157 and K-12. We also confirmed that the presence of the antibiotics used as selecting agents resulted in no statistically significant effect on the IS 629 excision frequencies. To determine whether the ECs1305-mediated enhancement of IS 629 excision is a process dependent on TPase activity, we constructed three reporter plasmids encoding mutant IS 629 TPases. In these mutants, one of the three acidic amino-acid residues constituting the DDE motif, which represents the active centre of the IS TPase [2] , was substituted with alanine (D244A, D303A and E339A). K-12 derivatives carrying a plasmid-encoded ECs1305 and the plasmids expressing these mutant TPases exhibited no IS 629 excision ( Supplementary Fig. S1 ). This result indicates that the ECs1305-mediated enhancement of IS 629 excision requires an active IS 629 TPase. To determine whether other host factors are also involved in the excision of IS 629 by ECs1305, we constructed a series of O157 Sakai mutants in which genes encoding host factors that have been demonstrated or suggested to be involved in the regulation of Tn transposition or TPase-independent IS deletion were deleted ( Supplementary Fig. S2a ). These gene products may be involved in the transposition or deletion of IS elements at various levels, such as the expression of TPase genes, transpososome assembly, replication slippage or DNA repair (see refs 2 , 21 for reviews). Because we were unable to delete the hns , dam and recB genes in O157 Sakai, we constructed deletion mutants for these three genes from GMEC101, a K-12 derivative containing a chromosomally inserted ECs1305 ( Supplementary Fig. S2b ). Many of these deleted genes affected ECs1305-mediated IS 629 excision in various ways ( Supplementary Fig. S2 ). However, the increase or decrease of the IS 629 excision frequency induced by the deletion of these genes was only marginal (at most, ∼ 50-fold) compared with the effect of ECs1305 deletion (>10 6 -fold decrease). Thus, the roles of these host factors in the observed IS 629 excision are minor or indirect. For example, the excision frequency slightly increased in the absence of host factors, which would be expected to affect the stability of ECs1305 and/or IS TPase (the ClpXP protease) or their gene expression (the H-NS protein). The frequency of IS 629 excision decreased in a mutant lacking HU, which is a histone-like protein that may assist in transpososome assembly or in other processes requiring higher-order DNA structures. Some reduction was also observed for the excision frequency in mutants lacking RecA, B or C proteins, suggesting that DNA repair processes mediated by these proteins contribute only slightly to the observed IS 629 excision. Taken together, our results indicate that ECs1305 has an essential role in high-frequency IS 629 excision in an IS TPase-dependent manner, although it is possible that some unknown host factor(s) is(are) also required for the process. Therefore, we designated ECs1305 as an IS-excision enhancer (IEE). IEE-promoted IS excision induces various genomic deletions We next examined whether IEE actually promotes the excision of IS 629 copies in the O157 Sakai genome using a multiplex PCR-based method (the IS-printing method) that we recently developed for O157 strain typing [22] . Using this method, most of the IS 629 copies in the O157 Sakai genome can be detected by production of a ladder band pattern using two sets of multiplex PCR primers (the first and second sets in Fig. 2a–d ), each comprising an IS 629 inside primer and multiple primers targeted to the flanking regions for each IS 629 element. Two IS 629 copies that are not included in the IS-printing system were examined using a similar system (the third set in Fig. 2a–d ). Thus, we were able to detect structural alterations occurring at any of the IS 629 insertion sites in the O157 Sakai genome (that is, deletion of IS 629 and/or flanking regions) by inspecting the ladder patterns ( Fig. 2a–d ). After O157 Sakai cells possessing both the IS 629 TPase- and the IEE-expressing plasmids were cultivated for 24 h in Luria-Bertani (LB) broth containing L -arabinose to induce IEE expression, 32 single colonies (referred to as Ex06001–Ex06032) were randomly selected and analysed by the IS-printing method. Alterations of the ladder pattern were detected in 29 clones (91%) in which 1–7 bands disappeared ( Fig. 2a ). Among the 30 bands, all but 5 that were derived from truncated IS 629 copies (IS629-4, -10, -p1, -pC and -pD) were found to be missing in one or more clones ( Fig. 2e ). No such alteration in the ladder pattern occurred in O157 Sakai cells containing either the TPase- or the IEE-expressing plasmid alone ( Fig. 2b–d ). This indicates that IEE, TPase and an IS 629 sequence with a complete TIR recognized by TPase in transposition [2] are required for IEE-induced structural alterations. Notably, none of the O157 Sakai genomic regions containing 19 other types of IS elements (not IS 629 ) with complete TIRs underwent structural changes among the 32 clones ( Supplementary Fig. S3 ). 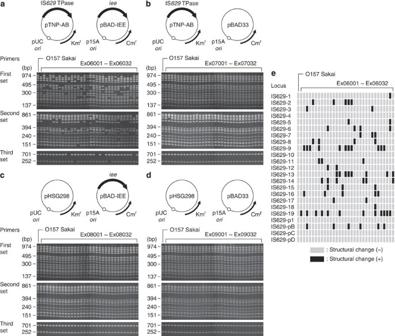Figure 2: IS629TPase- and IEE-induced structural alterations of IS629insertion sites in the O157 Sakai genome. Results of IS-printing analyses of the four sets of O157 Sakai derivatives (32 clones each) that were obtained after overexpression of IS629TPase and IEE together (a), IS629TPase alone (b), IEE alone (c) or neither IS629TPase nor IEE (d) are shown. Structures of the IS629TPase expression plasmid (pTNP-AB), the IEE expression plasmid (pBAD-IEE) and their control plasmids that were used for overexpression are also shown. Ex06001–Ex06032, Ex07001–Ex07032, Ex08001–Ex08032 and Ex09001–Ex09032 indicate the clone numbers in each set of the O157 Sakai derivatives. IS-printing analysis was performed using three sets of multiplex PCR primers (the first to third sets). All 23 IS629insertion sites in the O157 Sakai genome were examined by multiplex PCR followed by agarose gel electrophoresis. The presence or absence of structural alterations at each IS629insertion site was determined according to the ladder band patterns observed for each clone. (e) The results of IS-printing analysis of clones Ex06001–Ex06032 shown in panel (a) are summarized. Grey and black rectangles indicate IS629insertion sites without and with structural changes, respectively. Figure 2: IS 629 TPase- and IEE-induced structural alterations of IS 629 insertion sites in the O157 Sakai genome. Results of IS-printing analyses of the four sets of O157 Sakai derivatives (32 clones each) that were obtained after overexpression of IS 629 TPase and IEE together ( a ), IS 629 TPase alone ( b ), IEE alone ( c ) or neither IS 629 TPase nor IEE ( d ) are shown. Structures of the IS 629 TPase expression plasmid (pTNP-AB), the IEE expression plasmid (pBAD-IEE) and their control plasmids that were used for overexpression are also shown. Ex06001–Ex06032, Ex07001–Ex07032, Ex08001–Ex08032 and Ex09001–Ex09032 indicate the clone numbers in each set of the O157 Sakai derivatives. IS-printing analysis was performed using three sets of multiplex PCR primers (the first to third sets). All 23 IS 629 insertion sites in the O157 Sakai genome were examined by multiplex PCR followed by agarose gel electrophoresis. The presence or absence of structural alterations at each IS 629 insertion site was determined according to the ladder band patterns observed for each clone. ( e ) The results of IS-printing analysis of clones Ex06001–Ex06032 shown in panel ( a ) are summarized. Grey and black rectangles indicate IS 629 insertion sites without and with structural changes, respectively. Full size image We further analysed the structures of all IS 629 insertion sites that underwent structural alterations (78 sites in 29 clones, Supplementary Fig. S4 ) and found that various types of genomic deletions were generated by IEE and IS 629 TPase. As summarized in Fig. 3 , these genomic deletions were categorized into four types: (I) deletion of IS 629 with an adjacent short sequence of 1–7 bp (mainly 3 or 4 bp); (II) deletion of IS 629 with an adjacent long sequence; (III) partial deletion of IS 629 ; and (IV) deletion of a long sequence adjacent to IS 629 . In types I, II and III, additional deletion of a 3–5 bp sequence (mainly 3 bp) located adjacent to the other end of IS 629 was also sometimes observed (types Ib, IIb and IIIb in Fig. 3 ). 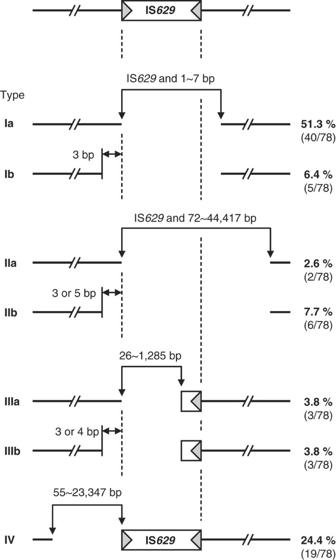Figure 3: Various genomic deletions generated by IEE in the presence of IS629TPase. Structural changes of IS629insertion sites in the O157 Sakai genome that were induced by IEE in the presence of IS629TPase were classified into four types. In types I and II, the entire IS629sequence was deleted, together with short (1–7 bp, mainly 3 or 4 bp) and long (72–44,417 bp) adjacent sequences, respectively. In type III, portions (26–1,285 bp) of the 1,310-bp IS629sequence were deleted. Deletion occurred at one IS end in types Ia, IIa and IIIa, and additional deletions of adjacent sequences occurred at the other IS end in types Ib, IIb and IIIb. In type IV, only the genomic segments adjacent to IS629(55–23,347 bp) were deleted without deletion of the IS element. Grey triangles indicate TIRs of IS629. The detection frequency of each type is expressed in percentage and the number of clones obtained for each type is indicated in parenthesis. Figure 3: Various genomic deletions generated by IEE in the presence of IS 629 TPase. Structural changes of IS 629 insertion sites in the O157 Sakai genome that were induced by IEE in the presence of IS 629 TPase were classified into four types. In types I and II, the entire IS 629 sequence was deleted, together with short (1–7 bp, mainly 3 or 4 bp) and long (72–44,417 bp) adjacent sequences, respectively. In type III, portions (26–1,285 bp) of the 1,310-bp IS 629 sequence were deleted. Deletion occurred at one IS end in types Ia, IIa and IIIa, and additional deletions of adjacent sequences occurred at the other IS end in types Ib, IIb and IIIb. In type IV, only the genomic segments adjacent to IS 629 (55–23,347 bp) were deleted without deletion of the IS element. Grey triangles indicate TIRs of IS 629 . The detection frequency of each type is expressed in percentage and the number of clones obtained for each type is indicated in parenthesis. Full size image Among the four types of deletions, the most frequently generated was type Ia (51.3%), which corresponds to precise or simple excision. In the transposition process of IS 3 family members, TPases first cleave one DNA strand at the 3′ end of the IS element [7] , [23] ( Fig. 4a ), and the liberated 3′ end is transferred to the same DNA strand at a position 3 or 4 bp away from the 5′ end of the IS element to generate a figure-eight intermediate ( Fig. 4b,c ). In the final step, DNA replication from the figure-eight junction generates a circular transposition intermediate and regenerates the donor DNA containing the original IS copy [2] , [24] . IEE probably functions in this last step to guide the process towards deleting the IS 629 copy from the donor DNA ( Fig. 4d ). Although the molecular mechanism of this phenomenon has yet to be clarified, second-strand cleavage and resealing of donor DNA seem to be required for IS 629 deletion. In several cases, deletion of 1, 5, 6 or 7 bp of the adjacent sequence was also observed. These atypical deletions may have been generated by imprecise strand transfer. 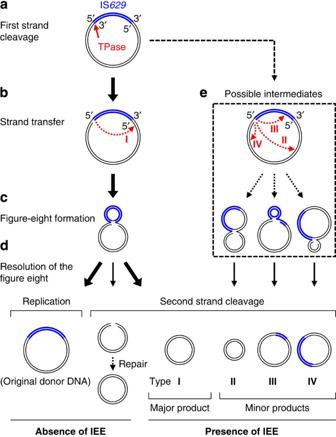Figure 4: Possible pathways for IS629excision and for the generation of various types of genomic deletions on IS excision. Although the process of IS629transposition has not been characterized, it is most likely that it transposes in a process similar to that of other IS3family members7. (a) TPase first cleaves one strand at the 3′ end of IS629(thick blue line) as indicated by the red arrow. (b) The liberated 3′ end is transferred to the proximity of the 5′ end of IS629(usually 3 or 4 bp away from the 5′ end) on the same strand, as indicated by the dotted red arrow I. (c) The strand transfer event generates a figure-eight structure in which the ends of IS629are joined by a single-stranded bridge. (d) DNA replication from the figure-eight junction generates a circular transposition intermediate and regenerates the donor DNA containing the IS copy. It is unknown whether liberation of the circle by some other mechanism(s), such as second-strand cleavage, occurs in the normal transposition process. If this does happen, the ends of the linearized donor DNA would need to be repaired for its survival. In the presence of IEE, various types of genomic deletions occur at IS insertion sites. The major product is a type I deletion representing simple excision, and other types of genomic deletions (types II, III and IV) are minor products. (e) If aberrant strand transfer (to a genome position far away from the 5′ end of IS629, inside of IS629, or very far from the 5′ end (that is, near the 3′ end of IS629, where the first strand cleavage occurred)) occurred, as indicated by dotted arrows II, III and IV, they would be intermediates for the formation of each variant type of genomic deletion. Figure 4: Possible pathways for IS 629 excision and for the generation of various types of genomic deletions on IS excision. Although the process of IS 629 transposition has not been characterized, it is most likely that it transposes in a process similar to that of other IS 3 family members [7] . ( a ) TPase first cleaves one strand at the 3′ end of IS 629 (thick blue line) as indicated by the red arrow. ( b ) The liberated 3′ end is transferred to the proximity of the 5′ end of IS 629 (usually 3 or 4 bp away from the 5′ end) on the same strand, as indicated by the dotted red arrow I. ( c ) The strand transfer event generates a figure-eight structure in which the ends of IS 629 are joined by a single-stranded bridge. ( d ) DNA replication from the figure-eight junction generates a circular transposition intermediate and regenerates the donor DNA containing the IS copy. It is unknown whether liberation of the circle by some other mechanism(s), such as second-strand cleavage, occurs in the normal transposition process. If this does happen, the ends of the linearized donor DNA would need to be repaired for its survival. In the presence of IEE, various types of genomic deletions occur at IS insertion sites. The major product is a type I deletion representing simple excision, and other types of genomic deletions (types II, III and IV) are minor products. ( e ) If aberrant strand transfer (to a genome position far away from the 5′ end of IS 629 , inside of IS 629 , or very far from the 5′ end (that is, near the 3′ end of IS 629 , where the first strand cleavage occurred)) occurred, as indicated by dotted arrows II, III and IV, they would be intermediates for the formation of each variant type of genomic deletion. Full size image The generation of other types of deletion was an unexpected finding. All these variant types were, however, formed only when IEE and the IS 629 TPase were coexpressed ( Fig. 2 ), indicating that they were generated in a process coupled with IS excision mediated by IEE and the IS 629 TPase. Indeed, none of these variant deletion types were detected in the reporter plasmid assay ( Fig. 1a ), in which only precise excision was detectable. Notably, all of these variant deletions were observed in naturally occurring O157 strains [14] . The mechanism(s) to generate these types of deletion is(are) unknown at present. It is also unknown why type IV deletions were generated at a relatively high frequency (24.4%). It may be possible to assume that they were generated by aberrant strand transfer ( Fig. 4e ), but this requires future examination. It is also important to note that IEE mainly induced the removal of IS 629 from the genome (75.6% of the structural changes). The result of Southern blot analysis of the 32 clones (Ex06001–Ex06032) using an IS 629 -specific probe indicated that the total copy number of IS 629 decreased in most clones ( Fig. 5 ). Several new signals that were absent from the parent strain were detected in several clones, but many of these were probably generated by type III or IV deletions. 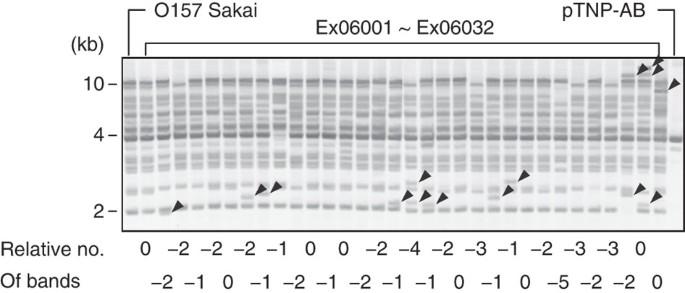Figure 5: Southern hybridization analysis of O157 Sakai and clones Ex06001–Ex06032 using an IS629-specific probe. To determine the difference in the total number of IS629copies in clones Ex06001–Ex06032, Southern hybridization analysis using an IS629-specific probe was performed.SspI-digested genomic DNA was separated by pulsed-field gel electrophoresis and subjected to Southern hybridization analysis. The DNA probe used was derived from the central part (positions 308–607) of IS629. The differences in the total copy number deduced for each clone (relative to that of the parent strain O157 Sakai) are indicated at the bottom. Signals that are detected in each clone but not in the parent strain are indicated by arrows. Only pTNP-AB plasmid DNA was applied to the lane labelled pTNP-AB. Note that the total copy number did not increase in any of the 32 clones. Figure 5: Southern hybridization analysis of O157 Sakai and clones Ex06001–Ex06032 using an IS 629 -specific probe. To determine the difference in the total number of IS 629 copies in clones Ex06001–Ex06032, Southern hybridization analysis using an IS 629 -specific probe was performed. Ssp I-digested genomic DNA was separated by pulsed-field gel electrophoresis and subjected to Southern hybridization analysis. The DNA probe used was derived from the central part (positions 308–607) of IS 629 . The differences in the total copy number deduced for each clone (relative to that of the parent strain O157 Sakai) are indicated at the bottom. Signals that are detected in each clone but not in the parent strain are indicated by arrows. Only pTNP-AB plasmid DNA was applied to the lane labelled pTNP-AB. Note that the total copy number did not increase in any of the 32 clones. Full size image Effect of IEE on other types of IS elements Using a reporter plasmid-based assay systems similar to that shown in Figure 1a , we examined whether IEE promotes the excision of other types of IS elements: two other IS 3 family members (IS 2 and IS 3 ) and six IS elements each belonging to different families (IS 1 , IS 4 , IS 5 , IS 26 , IS 30 and IS 621 ; Fig. 6 ). The excision of IS 2 and IS 3 was promoted by IEE to the same level as that for IS 629 , suggesting that the IS excision-enhancing activity of IEE may cover the entire IS 3 family. Among the other IS elements, the excision frequencies of IS 1 and IS 30 also clearly increased in the presence of IEE, although to a lesser extent compared with that of the IS 3 family. Thus, IEE enhances the excision of (minimally) members of the IS 3 , IS 1 and IS 30 families. Although it is unknown whether a figure-eight intermediate is formed during IS 1 transposition, IS 30 has been shown to form this structure [25] . This raises the possibility that IEE may function on a wide range of IS elements that transpose through the formation of figure-eight intermediates. 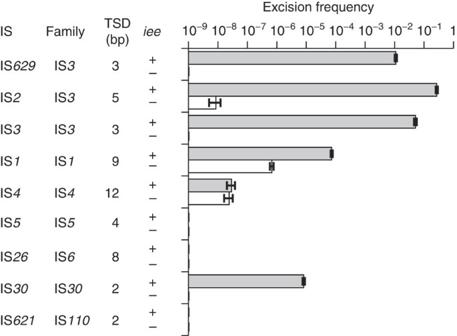Figure 6: Excision frequencies of various IS elements in the presence or absence of IEE. Excision frequencies of IS1, IS2, IS3, IS4, IS5, IS26, IS30and IS621in the presence or absence of IEE were examined in K-12 using reporter plasmids similar to pDN-TcR but comprising a cognate TPase coding region and TIR regions. The excision frequency was determined by dividing the number of ampicillin-resistant (Apr) colonies by tetracycline-resistant (Tcr) colonies (mean±s.d.,n=3). The IS family to which each IS belongs and the lengths of target site duplication (TSD) generated by each IS are indicated according to the descriptions in ISfinder5(http://www-is.biotoul.fr/). Plus and minus symbols indicate the presence and absence, respectively, of theieegene on the additional plasmid. The difference of the excision frequencies of IS4(pIEE1+) and IS4(pIEE1−) was not statistically significant (P<0.01). No Aprcolony was obtained for IS629(pIEE1−), IS3(pIEE1−), IS5(pIEE1+/−), IS26(pIEE1+/−), IS30(pIEE1−) or IS621(pIEE1+/−). Figure 6: Excision frequencies of various IS elements in the presence or absence of IEE. Excision frequencies of IS 1 , IS 2 , IS 3 , IS 4 , IS 5 , IS 26 , IS 30 and IS 621 in the presence or absence of IEE were examined in K-12 using reporter plasmids similar to pDN-TcR but comprising a cognate TPase coding region and TIR regions. The excision frequency was determined by dividing the number of ampicillin-resistant (Ap r ) colonies by tetracycline-resistant (Tc r ) colonies (mean±s.d., n =3). The IS family to which each IS belongs and the lengths of target site duplication (TSD) generated by each IS are indicated according to the descriptions in ISfinder [5] ( http://www-is.biotoul.fr/ ). Plus and minus symbols indicate the presence and absence, respectively, of the iee gene on the additional plasmid. The difference of the excision frequencies of IS 4 (pIEE1+) and IS 4 (pIEE1−) was not statistically significant ( P <0.01). No Ap r colony was obtained for IS 629 (pIEE1−), IS 3 (pIEE1−), IS 5 (pIEE1+/−), IS 26 (pIEE1+/−), IS 30 (pIEE1−) or IS 621 (pIEE1+/−). Full size image It is noteworthy that the effect of IEE on IS 1 was significantly less pronounced than that on IS 3 family members and IS 30 . This phenomenon may be related to the finding that IS 1 appears to be able to use two pathways for transposition [26] : one involves excision of a circular transposition intermediate (similar to the IS 3 family) and thus would be expected to be IEE sensitive, whereas the other involves cointegrate formation and would not be sensitive to IEE. Wide distribution of IEE homologues and their phylogenies The iee gene is located in a large integrative element, SpLE1, in O157 EHEC and in SpLE1-like elements in O26, O111 and O103 EHECs. These mobile genetic elements are specifically distributed in these EHEC strains [27] ( Supplementary Fig. S5 ), and the iee gene is not present in other sequenced E. coli strains, with the single exception of strain ED1a (ref. 28 ). Thus, IEE shows a strain-specific distribution in E. coli . In ED-1, a commensal E. coli strain, the iee gene is located in a different type of genetic element that has been integrated into a tRNA gene ( thrW ) ( Supplementary Fig. S5 ). A BLASTP search of the GenBank NR database with filtering of results by hit-length coverage (>80%) and sequence identity (>30%) identified many IEE homologues from a broad range of bacteria. 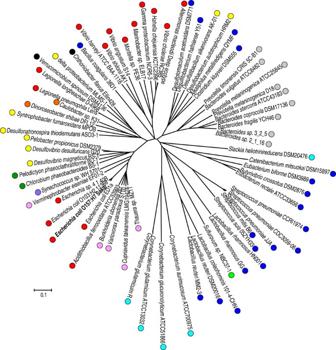Figure 7: Phylogeny of IEE homologues. IEE homologues were identified by a BLASTP search of the GenBank NR database with filtering of the results by hit-length coverage (>80%) and sequence identity (>30%). Amino-acid sequences of the IEE homologues were aligned using CLUSTALW in MEGA4 software49, and a neighbour-joining tree was generated with a bootstrap of 1,000 replicates. The names of the bacterial species and strains in which each homologue was discovered are shown. The phylum (or class) of the species is indicated by coloured circles: orange,Alphaproteobacteria; pink,Betaproteobacteria; red,Gammaproteobacteria; yellow,Deltaproteobacteria; light green,Epsilonproteobacteria; grey,Bacteroides; green,Chlorobi; violet,Cyanobacteria; blue,Firmicutes; light blue,Actinobacteria; and black,Verrucomicrobia. The size bar represents the number of substitutions per site. The IEE homologues from different phyla often cluster together, indicating that the evolution of the IEE homologues did not follow that of their host genomes. Phylogenetic analysis of these IEE homologues revealed that the homologues from different phyla often cluster together ( Figure 7 ; different phyla are indicated by circles of different colour). This finding indicates that the evolution of IEE homologues did not follow that of the host genomes. Furthermore, the distribution of IEE homologues suggests that they have spread in each species in a strain-specific manner, as observed in E. coli . For example, among the four fully sequenced Legionella pneumophila strains, IEE homologues were found in only two. In Bacteroides fragilis , Desulfitobacterium hafniense , Lactobacillus rhamnosus and Streptococcus pneumoniae as well, IEE homologues were found only in one strain among the two or more sequenced strains. In these five species, genes for their IEE homologues were located in strain-specific regions or genomic islands ( Supplementary Fig. S6 ). Figure 7: Phylogeny of IEE homologues. IEE homologues were identified by a BLASTP search of the GenBank NR database with filtering of the results by hit-length coverage (>80%) and sequence identity (>30%). Amino-acid sequences of the IEE homologues were aligned using CLUSTALW in MEGA4 software [49] , and a neighbour-joining tree was generated with a bootstrap of 1,000 replicates. The names of the bacterial species and strains in which each homologue was discovered are shown. The phylum (or class) of the species is indicated by coloured circles: orange, Alphaproteobacteria ; pink, Betaproteobacteria ; red, Gammaproteobacteria ; yellow, Deltaproteobacteria ; light green, Epsilonproteobacteria ; grey, Bacteroides ; green, Chlorobi ; violet, Cyanobacteria ; blue, Firmicutes ; light blue, Actinobacteria ; and black, Verrucomicrobia . The size bar represents the number of substitutions per site. The IEE homologues from different phyla often cluster together, indicating that the evolution of the IEE homologues did not follow that of their host genomes. Full size image These results suggest that IEE homologues have been spread to a variety of bacteria strains by horizontal gene transfer. To gain further insight into this issue, we analysed the genomic locations of all the other 24 IEE homologues that were identified in bacteria species, of which only a single strain has so far been fully sequenced ( Supplementary Fig. S7 ). Among the homologues analysed, many (at least 19 of 24) were encoded in genomic regions exhibiting low GC content and/or containing genes related to mobile elements, such as phage, Tn or IS. Furthermore, two additional IEE homologues were found on plasmids ( Dinoroseobacter shibae strain DFL12 and Caulobacter sp . strain K31). These results support the notion that IEE homologues have been spread widely in bacteria by horizontal gene transfer. The identification of many IEE homologues allowed us to perform multiple sequence alignment analysis ( Supplementary Fig. S8 ). From this analysis, we found four regions that are highly conserved between the IEE family of proteins (regions 1–4). A domain search using SMART [29] and Pfam [30] revealed that regions 1 and 2 exhibit some similarity to a sequence motif found in eukaryotic/archaeal primases (pfam01896), whereas regions 3 and 4 contain a DEXDc motif (pfam00270) and a HELICc motif (smart00490), respectively, which are found in protein families such as the DEAD and DEAH box helicases. Although the relationship between IEE function and these motifs must be elucidated in future, our preliminary results indicate that alanine substitution of several invariant amino-acid residues found in regions 3 and 4 considerably reduces IEE activity to promote IS 629 excision. In this study, we showed that IEE promotes the excision of IS elements belonging to the IS 3 family, as well as those belonging to the IS 1 and IS 30 families, from bacterial genomes. Although the molecular mechanism of IEE action remains unknown, the identification of IEE is scientifically important from several perspectives. First, IEE is the first bacterial protein that has been shown to promote IS excision in a TPase or transposition-dependent manner; although it may not function directly on TPase, it may function on an intermediate generated during transposition. Several host factors, such as proteins for DNA repair and recombination, may also induce the deletion of Tns [31] but in a TPase-independent manner and at much lower efficiencies compared with that promoted by IEE ( Supplementary Fig. S2 ). This function of IEE is particularly important for bacterial cells because, unlike eukaryotic cells, most bacterial species have no specific end-joining activity to regenerate and protect the donor genome after IS excision. Second, IEE-mediated IS excision generates a variety of genomic deletions. IS elements and their transpositions are generally regarded as one of the major driving forces generating various genomic deletions, but precise mechanisms remain unknown for many of the genomic deletions detected in sequenced bacterial genomes. The action of IEE can explain how genomic deletions are generated on IS transposition or excision. Third, structural features of the donor DNA regenerated after IEE-induced IS excision, particularly for variant types of deletions, may provide further insight into the process of IS transposition. Processes leading to the generation of such variant types of genomic deletions may take place only when IEE is present. However, it is also possible that rare or aberrant intermediates that are unable to survive in the normal process of transposition (that is, in the absence of IEE) may be trapped by the action of IEE. If so, the structures of these IEE-induced deletions may represent or reflect the structures of rare intermediates generated in the normal transposition process. Finally, IEE can be regarded as a new type of genetic system that controls the copy number of Tns in host genomes. The invasion and proliferation of Tns are important in long-term genome evolution, but their uncontrolled proliferation is sometimes detrimental to the host. Thus, various genetic systems to suppress or attenuate their transposition activities have evolved. Tc 1 transposition is silenced by RNA interference in the Caenorhabditis elegans germ line [32] . This system also suppresses the transposition of other types of Tns, such as Tc 3 , Tc 5 and Tc 7 (ref. 33 ). Silencing of Tns is also achieved by epigenetic mechanisms through modification of histone tails, DNA methylation and chromatin remodelling [34] . In addition, the transposition activities of some Tns are negatively regulated by a repressor encoded by Tns themselves, as seen in the P element of Drosophila [35] and in several bacterial Tns, such as Tn 5 (ref. 36 ), IS 1 (refs 37 , 38 ) and members of the IS 3 family [39] . The coexpression of IEE and of IS 629 TPase reduced the copy number of IS 629 in O157, and this could happen to other members of the IS 3 family and to members of (minimally) the IS 1 and IS 30 families. This type of control mechanism has not been described in eukaryotes, archaea or bacteria. The identification of many IEE homologues from a broad range of bacterial species represents an important finding in terms of gene evolution. The results of the phylogenetic analysis of these IEE homologues indicate that their evolution did not follow that of their host genomes, instead suggesting the involvement of horizontal gene transfer in the spread of IEE homologues among bacteria. This idea is supported by the observation that IEE homologues from several bacterial species for which multiple genome sequences are available clearly show a strain-specific distribution, and many of the other IEE homologues are also encoded in genomic regions of apparently foreign origin. Thus, IEEs may represent a novel protein family that has been widely spread by horizontal gene transfer and has coevolved with a number of IS elements belonging to the IS 3 and other families. Further, these proteins may have pivotal roles in the evolution of many bacterial species or strains by inducing IS excision and various types of genomic deletions. Bacterial strains and culture conditions RIMD0509952 (referred to as O157 Sakai) is an EHEC O157:H7 strain isolated from a typical patient during the Sakai outbreak that occurred in Japan in 1996. MG1655 (referred to as K-12) is an E. coli K-12 strain maintained as a laboratory strain with minimal genetic manipulation. The genome sequences of both O157 Sakai and K-12 were previously determined [19] , [40] . The other EHEC O157, O26, O111 and O103 strains used for the analysis of excision frequencies ( Fig. 1b ) were also clinical isolates [41] , [42] . GMSS401 is an isogenic mutant of O157 Sakai in which ECs1305 was deleted from the chromosome. GMEC101 is an isogenic mutant of K-12 in which ECs1305 was inserted in an IS 3 copy on the chromosome. The isogenic mutants were generated using the method developed by Djafari et al . [43] All strains were grown in LB broth [44] supplemented, when necessary, with 50 μg ml −1 ampicillin (Ap), 30 μg ml −1 chloramphenicol (Cm), 20 μg ml −1 kanamycin (Km) or 20 μg ml −1 tetracycline (Tc). The selection of mutants was carried out on LB agar plates supplemented with the appropriate antibiotic(s). DNA manipulations Restriction endonucleases and T4 DNA ligase were purchased from Takara Bio. E. coli cells were transformed by electroporation [44] . Plasmid DNA was prepared using a QIAfilter Plasmid kit (Qiagen). Nucleotide sequences were determined by the dideoxy chain termination method [45] using a BigDye Terminator Cycle Sequencing kit and an Applied Biosystems 3130 sequencer (Applied Biosystems) according to the manufacturer's instructions. Construction of plasmids pDN-TcR was used as a reporter plasmid in the IS 629 excision assay ( Fig. 1a ). In this plasmid, IS 629 -Tc and the IS 629 TPase gene are inserted in the Ap r gene ( Sca I site) and the Hin cII site of pUC18, respectively [18] . IS 629 -Tc is an IS 629 analogue, in which the IS 629 TPase gene was replaced with the Tc r gene from pBR322 (ref. 18 ). pTNP-AB is an IS 629 TPase expression plasmid carrying a part of IS 629 comprising the −10 and −35 promoter region, the Shine–Dalgarno sequence and the TPase coding region [18] . The reporter plasmids for analysing other types of IS elements shown in Figure 6 were constructed by substituting the TPase coding region and the TIR regions of IS 629 in pDN-TcR with those of each cognate IS element. The TPase coding regions and the TIR regions of other IS elements were amplified by PCR using the primers listed in Supplementary Table S1 . The amplicons were then used as pairs of complementary primers in the PCR-based site-directed mutagenesis method [46] . PCR was performed in a 50 μl reaction mixture containing 50 ng of template DNA (pDN-TcR), 100 ng of amplicon, 0.2 mM of each deoxynucleoside triphosphate, PCR buffer and 1 U of KOD-plus DNA polymerase (Toyobo) with 18 cycles of 15 s at 94 °C, 30 s at 60 °C and 5.5 min at 68 °C. IS 1 , IS 2 and IS 3 have two consecutive and partially overlapping open reading frames (ORFs), orfA and orfB ( insA and insB for IS 1 ), positioned in the 0 and −1 phases, respectively. Because, as in IS 629 (ref. 17 ), the TPases of these IS elements are produced as a fused protein OrfAB (or InsAB′), by programmed frameshifting between the two ORFs [2] , a 1-bp insertion was introduced in the overlapping region of the two ORFs of IS 1 , IS 2 and IS 3 by PCR-based site-directed mutagenesis [46] using pairs of complementary primers IS1-SF and IS1-SR, IS2-SF and IS2-SR, and IS3-SF and IS3-SR, respectively ( Supplementary Table S1 ). pBAD-IEE is a plasmid in which ECs1305 (the iee gene) was inserted into the Sma I site of pBAD33 (ref. 47 ), and expression of the iee gene is induced by L -arabinose. The coding region of ECs1305 was amplified by PCR with two primers (5′-AGGAGGAATTCACCATGGTTCATAAATCTGACAGTGATGAATTAG-3′ and 5′-TCATTAAATCACTGATTCATCGCCGTCAGC-3′) and used for plasmid construction. PCR was performed in a 50 μl reaction mixture containing template DNA (genomic DNA of O157 Sakai), 0.3 μM each of the two primers, 0.2 mM of each deoxynucleoside triphosphate, PCR buffer and 1 U of KOD-plus DNA polymerase (Toyobo) with 25 cycles of 15 s at 94 °C, 30 s at 60 °C and 25 min at 68 °C. By nucleotide sequencing, we confirmed that no unexpected mutation was introduced into the cloned ECs1305 fragment. pBAD33 was provided by the National BioResource Project (NIG, Japan): E. coli . Analysis of structural alterations in IS 629 insertion sites O157 Sakai(pTNP-AB/pBAD-IEE), which is an O157 Sakai derivative containing both pTNP-AB and pBAD-IEE, was cultivated at 37 °C for 24 h in LB broth containing 0.2% L -arabinose to induce iee gene expression. The bacterial cells were then grown on an LB plate, and 32 single colonies were randomly selected (Ex06001–Ex06032). Structural alterations in all but two IS 629 insertion sites in the genomes of these 32 clones were analysed using the IS-printing kit (Toyobo) according to the manufacturer's instructions. The two IS 629 insertion sites were analysed using primers 5′-CAGT GGATGCCAATAAGCCAG-3′ and 5′-GAGACACAATGCCCATCCTTCG-3′, respectively. Similar analyses were performed for another three sets of O157 Sakai-derived clones (Ex07001–Ex07032, Ex08001–Ex08032 and Ex09001–Ex09032), which were derived from O157 Sakai(pTNP-AB/pBAD33), O157 Sakai(pHSG298/pBAD-IEE) and O157 Sakai(pHSG298/pBAD33), respectively. pHSG298 and pBAD33 were used as controls for pTNP-AB and pBAD-IEE, respectively. To determine the altered structures of each IS 629 insertion site, we amplified the genomic segments containing the IS 629 insertion site from Ex06001 to Ex06032 by PCR using primer sets for whole-genome PCR scanning (a long-range PCR-based genome comparison system developed by Ohnishi et al . [41] ), and determined the nucleotide sequences of IS 629 -flanking regions. PCR analysis of IS elements other than IS 629 All O157 Sakai genomic loci with insertion of intact IS elements other than IS 629 (non-IS 629 ) were examined by PCR using primers shown in Supplementary Table S2 . PCR was performed in a 50 μl reaction mixture containing template DNA (genomic DNA of O157 Sakai or clones Ex06001–Ex06032), 0.2 μM of each primer, 0.2 mM of each deoxynucleoside triphosphate, PCR buffer and 1.25 U of Ex Taq DNA polymerase (Takara Bio) with 35 amplification cycles of 30 s at 95 °C, 30 s at 60 °C and 4 min at 72 °C. Pulsed-field gel electrophoresis Pulsed-field gel electrophoresis was performed by clamped homogeneous electric field electrophoresis using a CHEFF DR III apparatus (Bio-Rad Laboratories). Genomic DNA of each strain was prepared by the method described by Akiba et al . [48] Genomic DNA in sliced plugs was digested with 30 U of Ssp I at 37 °C for 16 h. Electrophoresis was conducted in a 1% agarose gel in 0.5× Tris-borate-EDTA buffer at 14 °C at 6 V cm −1 for 10 h with a pulse time of 4 s. Southern blot hybridization analysis A digoxigenin (DIG)-labelled PCR product was used as a DNA probe. A 300-bp fragment covering the central part of IS 629 was amplified by PCR in a 100-μl reaction mixture containing template DNA (genomic DNA of the O157 Sakai strain), 0.2 μM each of two primers (5′-GCAGTAACGATATCCTTCGCCAGGC-3′ and 5′-CGTAACAACTGACGCCAGACTTTACGC-3′), 10 μl of PCR DIG Labeling Mix (Roche Diagnostics), PCR buffer and 1.25 U of Ex Taq DNA polymerase (Takara Bio) for 30 amplification cycles of 94 °C for 30 s, 60 °C for 30 s and 72 °C for 30 s. The electrophoresed DNA was blotted onto a Hybond-N+ charged nylon membrane (GE Healthcare) by the standard method [44] . The blotted membrane was then probed with the DIG-labelled PCR product. Prehybridization and hybridization were carried out at 68 °C using PerfectHyb hybridization solution (Toyobo), and after washes with buffer A (2× SSC with 0.1% SDS) and buffer B (0.1× SSC with 0.1% SDS), signals were detected using a DIG Nucleic Acid Detection kit (Roche Diagnostics) according to the manufacturer's instructions. Data deposition: The nucleotide sequence of pBAD-IEE has been deposited in DDBJ/EMBL/GenBank under accession number AB598835 . How to cite this article: Kusumoto, M. et al . Insertion sequence-excision enhancer removes transposable elements from bacterial genomes and induces various genomic deletions. Nat. Commun. 2:152 doi: 10.1038/ncomms1152 (2011).